A mitochondria-targeted inhibitor of cytochromecperoxidase mitigates radiation-induced death The risk of radionuclide release in terrorist acts or exposure of healthy tissue during radiotherapy demand potent radioprotectants/radiomitigators. Ionizing radiation induces cell death by initiating the selective peroxidation of cardiolipin in mitochondria by the peroxidase activity of its complex with cytochrome c leading to release of haemoprotein into the cytosol and commitment to the apoptotic program. Here we design and synthesize mitochondria-targeted triphenylphosphonium-conjugated imidazole-substituted oleic and stearic acids that blocked peroxidase activity of cytochrome c /cardiolipin complex by specifically binding to its haem-iron. We show that both compounds inhibit pro-apoptotic oxidative events, suppress cyt c release, prevent cell death, and protect mice against lethal doses of irradiation. Significant radioprotective/radiomitigative effects of imidazole-substituted oleic acid are observed after pretreatment of mice from 1 h before through 24 h after the irradiation. Despite having evolved from organisms adapted to massive irradiation during the early development of Earth's biosphere, the human body—with its abundance of water—is vulnerable to radiolysis by high-energy (ionizing) irradiation. Medical applications of irradiation critically consider this sensitivity of normal tissues, particularly in the use of total body exposure for bone marrow transplantation patients. However, in uncontrolled situations of exposure to radiation, such as during a terrorist attack, or the unavoidable radiation exposure of flight crews during extended space missions, the development of protective measures is lagging behind, and there is an immediate need for the stockpiling of safe and effective radioprotectors/radiomitigators. Acute radiation syndrome is associated with damage to the haematopoietic system and gastrointestinal tract due to massive cell loss in radiosensitive tissues occurring largely via apoptosis [1] , [2] , [3] . Along with radicals generated by radiolysis of water, the execution of mitochondria-mediated apoptosis is universally associated with the production of reactive oxygen species [4] , [5] . Therefore, development of radiomitigators/radioprotectors for biodefense applications and radiotherapy has mostly focused on nonspecific thiol-based antioxidants that have shown clinically insignificant results [6] , [7] , [8] . Recently, reactive oxygen species production has been identified as a required step in selective peroxidation of a mitochondria-specific phospholipid, cardiolipin (CL), whose oxidation products are essential for the outer membrane permeabilization and release of pro-apoptotic factors [4] , [9] . The catalyst of the peroxidation reaction is cytochrome c (cyt c ) that forms a high-affinity complex with CL exhibiting potent peroxidase activity towards polyunsaturated CLs [9] . In normal mitochondria, CL and cyt c are spatially separated: the former is confined almost exclusively to the inner mitochondrial membrane, whereas the latter is located in the intermembrane space [10] . Early in apoptosis, CL migrates from the inner to the outer mitochondrial membrane—a process likely facilitated by one of the four candidate mitochondrial proteins: scramblase-3, nucleoside diphosphate kinase, mitochondrial isoforms of creatine kinase and t-Bid [11] , [12] , [13] . Trans-membrane re-distribution of CL makes physical interaction of CL and cyt c possible resulting in the formation of cyt c /CL complexes [9] . Several previous studies have proposed that there are two types of interaction of cyt c with anionic phospholipids: an electrostatic interaction and a specific hydrophobic interaction. Whereas the electrostatic interaction is mainly driven by the charges between the protein and anionic lipids, the hydrophobic interaction involves the insertion of the lipid acyl chain in a hydrophobic channel present in the structure of cyt c . It has been shown that both interactions are essential for initiating the peroxidase activity of cyt c [9] leading to peroxidation of bound polyunsaturated molecular species of CL. Notably, accumulation of peroxidized CL is essential for the execution of the apoptotic program. Conversely, prevention of CL peroxidation leads to inhibition of apoptosis [14] . In the present study, we reason that the new 'pro-oxidant' enzymatic activity of cyt c /CL complexes represents a target for anti-apoptotic radioprotective drugs. Specifically, the peroxidase activity is due to CL-induced partial unfolding of the protein in the complex resulting in a 'loosened' liganding capacity of haem-iron by a distal Met 80 (ref. 15 ). We hypothesize that 'locking' of the haem-iron coordination bond with a strong ligand delivered through the hydrophobic channel to the immediate proximity of the haem catalytic site would block the peroxidase activity, inhibit CL peroxidation and prevent the progression of apoptosis. Indeed, we demonstrate that mitochondria-targeted 3-hydroxypropyl-triphenylphosphonium (TPP)-conjugated imidazole-substituted oleic acid ( TPP-IOA ) and stearic acid ( TPP-ISA ) exert strong specific liganding of haem-iron in cyt c /CL complex, effectively suppressing its peroxidase activity and CL peroxidation, thus preventing cyt c release and cell death, and protecting mice against lethal doses of irradiation. Molecular modelling and docking studies We have designed ( Fig. 1 ) and synthesized ( Supplementary Fig. S1 ) imidazole-substituted fatty acids and their esters—imidazole substituted oleic acid ( IOA ), stearic acid ( ISA ) ( Fig. 1a,b ), imidazole substituted methyl ester of oleic acid ( IEOA , Fig. 1c ) and imidazole substituted dodecanoic acid ( IDA ) ( Fig. 1d )—assuming that these compounds will interact with cyt c by providing the imidazole group as a sixth ligand to the haem. A similar strategy was used to inhibit the terminal oxidation of fatty acids by CYP4A1 (ref. 16 ). Molecular modelling and docking studies of partially unfolded cyt c showed that 18-carbon-long IOA and ISA ( Fig. 2a–c ) as well as IEOA ( Fig. 2d ) with the imidazole moiety 7-carbon atoms away from the terminal methyl group indeed positioned the heterocycle close to haem such that the nitrogen atom of imidazole was within 2.4 Å ( IOA ), 2.5 Å ( IEOA ) and 2.7 Å ( ISA ) from the haem-iron. A hydrophobic channel formed by the displacement of the Met 80 -containing loop in the partially unfolded cyt c structure stabilized the interaction ( Fig. 2b , coloured in yellow). Notably, the truncated derivative IDA , with the imidazole-moiety attached to the terminal CH 2 -group, this specific positioning was not achieved and the imidazole nitrogen was 6.9 Å away from the haem-iron ( Fig. 2e ). 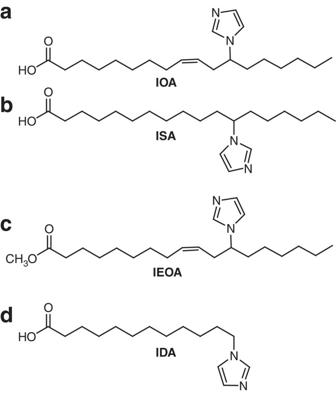Figure 1: Structural formulas of synthesized compounds. (a) 12-(1H-imidazol-1-yl)-(Z)-octadec-9-enoic acid (IOA); (b) 12-(1H-imidazol-1-yl)octadecanoic acid (ISA); (c) methyl 12-(imidazol-1-yl)-(Z)-octadec-9-enoate (IEOA); (d) 12-(imidazol-1yl)-dodecanoic acid (IDA). Synthetic and experimental details are provided inSupplementary Methods. Figure 1: Structural formulas of synthesized compounds. ( a ) 12-(1H-imidazol-1-yl)-(Z)-octadec-9-enoic acid ( IOA ); ( b ) 12-(1H-imidazol-1-yl)octadecanoic acid ( ISA ); ( c ) methyl 12-(imidazol-1-yl)-(Z)-octadec-9-enoate ( IEOA ); ( d ) 12-(imidazol-1yl)-dodecanoic acid ( IDA ). Synthetic and experimental details are provided in Supplementary Methods . 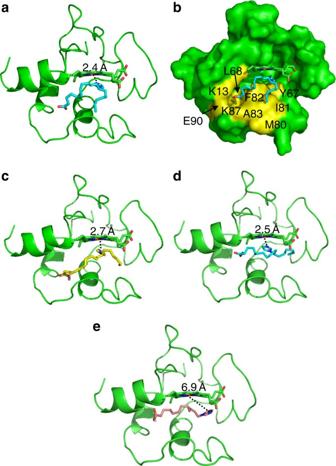Figure 2: Modelling of the binding of imidazole substituted fatty acids. (a,b)IOA, (c)ISA, (d)IEOA, and (e)IDA. Cytcis coloured in green and represented as cartoon in (a,c,d,e) and as surface in (b).IOA,IEOA,ISA,TPP-IOA,TPP-ISA,IDAand haem are represented as sticks.IOAandIEOAare coloured in cyan;ISAis coloured in yellow andIDAis coloured in wheat. The hydrophobic surface corresponding to the predicted IOA binding site is coloured in yellow (b). Full size image Figure 2: Modelling of the binding of imidazole substituted fatty acids. ( a , b ) IOA , ( c ) ISA , ( d ) IEOA , and ( e ) IDA . Cyt c is coloured in green and represented as cartoon in ( a , c , d , e ) and as surface in ( b ). IOA , IEOA , ISA , TPP-IOA , TPP-ISA , IDA and haem are represented as sticks. IOA and IEOA are coloured in cyan; ISA is coloured in yellow and IDA is coloured in wheat. The hydrophobic surface corresponding to the predicted IOA binding site is coloured in yellow ( b ). Full size image Suppression of peroxidase activity of cyt c complexes We next evaluated the effect of ISA , IOA and IEOA on the peroxidase activity of cyt c complexes with tetra-oleoyl-cardiolipin (TOCL) towards H 2 O 2 -driven oxidation of two prototypical phenolic substrates, Amplex Red ( Fig. 3a ) and etoposide ( Fig. 3b ). We found that ISA , IOA and IEOA acted as potent inhibitors of the peroxidase activity of cyt c /TOCL complexes with both substrates ( Fig. 3 ). Computer modelling showed that IOA ( Fig. 2a ), IEOA ( Fig. 2d ) and ISA ( Fig. 2c ) bind to cyt c in a similar fashion. The truncated derivative IDA , did not exert any inhibitory effect ( Fig. 3a ), in line with our computer modelling data. Because catalytic reactive intermediates of cyt c /CL peroxidase complexes—protein-immobilized (tyrosyl) radicals (Tyr • )—can be detected by electron paramagnetic resonance (EPR) spectroscopy [17] , we studied the effect of IEOA and IOA on H 2 O 2 -dependent formation of radicals ( Fig. 3c ). Both IOA and IEOA (but not IDA ) effectively quenched generation of Tyr • radicals. Finally, we assessed the ability of ISA and IEOA to inhibit peroxidase activity using isolated mouse liver mitochondria. To avoid decomposition of H 2 O 2 by catalase, we used tert -butyl hydroperoxide (tBOOH) as a source of oxidizing equivalents. Both ISA and IEOA suppressed peroxidase activity in a concentration-dependent manner ( Supplementary Fig. S2 ). 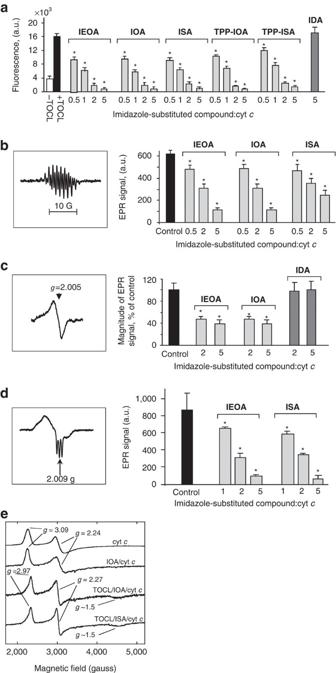Figure 3: Inhibition of peroxidase activity of cytc/TOCL complexes. (a) Assessments of peroxidase activity of cytc/TOCL by H2O2-induced oxidation of Amplex Red to resorufin. Data are means±s.d.,n=4, *P<0.01 (Student'st-test) versus control (TOCL/cytc/H2O2with noISAorIOAorIEOAorTPP-IOAorTPP-ISAadded). (b) A typical EPR spectrum of etoposide phenoxyl radicals (left panel). Assessments of peroxidase activity of cytc/TOCL by H2O2-induced oxidation of etoposide using EPR spectroscopy (right panel). (c) A typical low-temperature EPR spectrum of protein-immobilized (tyrosine) radicals (left panel). Assessments of protein-immobilized (tyrosine) radicals by low-temperature (77 K) EPR spectroscopy (right panel). (d)ISAandIEOAlimit accessibility of haem to small molecules. A typical low-temperature (77 K) EPR spectrum of cytc/TOCL complexes in the presence of Angeli's salt (left panel). Effects ofISAandIEOAon haem-nitrosylation of cytc/TOCL induced by nitroxyl (HNO) generated from Angeli's salt (right panel). Data are means±s.d.,n=3, *P<0.05 versus control (noISAandIEOAadded). (e) Liquid-He EPR evidence for ligation change in cytchaem-iron. X-band liquid-He (20 K) EPR spectra of cytc. Figure 3: Inhibition of peroxidase activity of cyt c /TOCL complexes. ( a ) Assessments of peroxidase activity of cyt c /TOCL by H 2 O 2 -induced oxidation of Amplex Red to resorufin. Data are means±s.d., n =4, * P <0.01 (Student's t -test) versus control (TOCL/cyt c /H 2 O 2 with no ISA or IOA or IEOA or TPP-IOA or TPP-ISA added). ( b ) A typical EPR spectrum of etoposide phenoxyl radicals (left panel). Assessments of peroxidase activity of cyt c /TOCL by H 2 O 2 -induced oxidation of etoposide using EPR spectroscopy (right panel). ( c ) A typical low-temperature EPR spectrum of protein-immobilized (tyrosine) radicals (left panel). Assessments of protein-immobilized (tyrosine) radicals by low-temperature (77 K) EPR spectroscopy (right panel). ( d ) ISA and IEOA limit accessibility of haem to small molecules. A typical low-temperature (77 K) EPR spectrum of cyt c /TOCL complexes in the presence of Angeli's salt (left panel). Effects of ISA and IEOA on haem-nitrosylation of cyt c /TOCL induced by nitroxyl (HNO) generated from Angeli's salt (right panel). Data are means±s.d., n =3, * P <0.05 versus control (no ISA and IEOA added). ( e ) Liquid-He EPR evidence for ligation change in cyt c haem-iron. X-band liquid-He (20 K) EPR spectra of cyt c . Full size image Liganding of haem-iron in cyt c /TOCL complexes To address whether ISA and IEOA act as strong ligands of haem-iron in cyt c /TOCL complexes, we used low-temperature EPR spectroscopy [18] . In the reduced form, cyt c /TOCL binds NO • to produce haem-nitrosylated complexes with characteristic EPR spectra [9] . Indeed, at 77 K, typical spectra of penta-, and hexa-coordinated cyt c were detectable on incubation of cyt c /TOCL complexes in the presence of a source of nitroxyl (HNO), Angeli's salt ( Fig. 3d ). ISA and IEOA ( Fig. 3d ) caused a concentration-dependent decrease of the EPR signal. To provide evidence for coordination changes of the haem-iron in cyt c , we performed liquid-He EPR measurements. The X-band EPR spectrum of native ferri-cyt c at pH 7.4, recorded at 20 K, exhibited anisotropic, low-spin signals, with g z =3.09, g y =2.24 and g x ~1 (usually unobserved) ( Fig. 3e ) indicative of His/Met axial coordination at the haem [19] , [20] . On the addition of IOA , there was no change in the EPR spectrum indicating retention of the native His/Met axial coordination ( Fig. 3e ). However, when IOA was added to the cyt c /TOCL complex, the EPR spectrum revealed the presence of another low-spin species ( g z =2.97, g y =2.27, g x ~1.5, Fig. 3e ) with g -values entirely consistent with His/imidazole coordination [20] , [21] . This signal was broadened on the low-field side, suggesting a combination of the native ferri-cyt c and a His/imidazole form. Spectral simulations (not shown) confirm an ~50:50 mixture of the native structure and the form in which Met 80 has been replaced by the imidazole moiety of IOA . These were the only signals observed; in particular, there were none at g ~6, indicating the absence of any penta- or hexacoordinate high-spin species. Similarly, ISA was able to change haem-iron coordination in cyt c , whereby Met 80 was substituted by the imidazole moiety ( Fig. 3e ). These results confirm experimentally that the imidazole moiety of imidazole fatty acids can indeed serve as a coordinating ligand for the haem substituting for Met 80 ligation. Inhibition of apoptosis by TPP-ISA and TPP-IOA We then explored the ability of imidazole substituted fatty acids to inhibit apoptosis in cells. To target imidazole substituted fatty acids into mitochondria, we esterified them with TPP-derived propanol ( Fig. 4a,b ), an organic cationic alcohol with delocalized electron density—known to be effectively 'electrophoresed' because of the negative potential on the inside of the organelle's membrane [22] . By using computer modelling, we confirmed that conjugation of ISA and IOA with TPP did not significantly affect their positioning within the immediate proximity of the cyt c 's haem-iron, that is, the nitrogen atom of the imidazole of both TPP-IOA and TPP-ISA was within 2.9 Å from the haem-iron ( Fig. 4c,d ). Moreover, TPP-ISA and TPP-IOA were as effective as non-conjugated ISA and IOA in inhibiting peroxidase activity of cyt c /TOCL complexes ( Fig. 3 ). 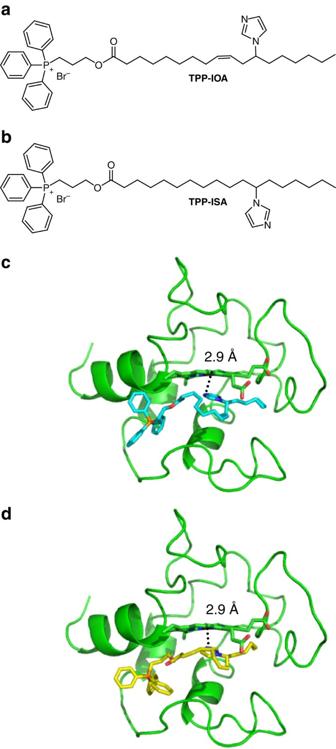Figure 4: Structures and molecular modelling ofTPP-IOAandTPP-ISA. (a,c) 9-(Z)-(3-((12-imidazol-1-yl)octadeca-9-enoyloxy)propyl)triphenylphosphonium bromide (TPP-IOA); (b,d) (3-(12-imidazol-1-yl)-octadecanoyl)propyl)triphenylphosphonium bromide (TPP-ISA);TPP-IOAis coloured in cyan,TPP-ISAis coloured in yellow. Figure 4: Structures and molecular modelling of TPP-IOA and TPP-ISA . ( a , c ) 9-(Z)-(3-((12-imidazol-1-yl)octadeca-9-enoyloxy)propyl)triphenylphosphonium bromide ( TPP-IOA ); ( b , d ) (3-(12-imidazol-1-yl)-octadecanoyl)propyl)triphenylphosphonium bromide ( TPP-ISA ); TPP-IOA is coloured in cyan, TPP-ISA is coloured in yellow. Full size image We further estimated the amounts of accumulated TPP-IOA in mitochondria of mouse embryonic cells using high-performance liquid chromatography (HPLC) and electrospray ionization mass spectrometry (ESI-MS) ( Supplementary Fig. S3 ). We found that most of TPP-IOA was present in mitochondria ( Supplementary Fig. S3 ). Assuming that the volume of mitochondria constitutes ~15–25% of the total volume of a cell, the mitochondrial enrichment factor becomes even greater such that the concentration of TPP-IOA in mitochondria may be as high as ~5 mM. It is likely that endogenous esterases can hydrolyse the ester-bond and release IOA and TPP-derived Propanol. To test this, we performed assessments of esterase activity of mitochondria and cytosolic fractions isolated from mouse embryonic cells based on HPLC measurements of TPP-IOA ( Supplementary Fig. S3 ). We found that hydrolysis of TPP-IOA takes place in both mitochondria and the cytosol. The hydrolysis rate in mitochondria was comparable to that in the cytosolic fraction ( Supplementary Fig. S3 ). Thus, both TPP-IOA and its de-esterifed form, IOA , could be present in mitochondria of mouse embryonic cells. Because TPP-conjugated imidazole-substituted fatty acids effectively partition into mitochondria, we examined whether they affected bioenergetic functions, particularly ATP production. Neither TPP-IOA nor TPP-ISA had any effect on ATP levels in mouse embryonic cells. Normally, mitochondria are the major source of superoxide radicals in mouse embryonic cells [23] , [24] . Assessments of intracellular superoxide production using dihydroethidium showed that neither TPP-IOA nor TPP-ISA had any effect on superoxide production in cells with or without radiation treatment ( Supplementary Fig. S4 ). For the anti-apoptotic action, it is essential that proposed haem-iron ligation is effective in inhibiting peroxidation of polyunsaturated species of CL. Therefore, we used an oxidizable tetra-linoleoyl-cardiolipin (TLCL), and conducted experiments on its cyt c /H 2 O 2 -induced oxidation ( Fig. 5 ). In the presence of H 2 O 2 , we detected accumulation of characteristic TLCL peroxidation products with multiple oxygenated linoleic acid residues detectable by ESI-MS ( Fig. 5a ). We found that both TPP-IOA and TPP-ISA inhibited cyt c /H 2 O 2 -induced oxidation of TLCL in a concentration-dependent manner. No difference in inhibition of TLCL oxidation between TPP-IOA and TPP-ISA was detected. The oxidation of TLCL was completely blocked at a ratio of cyt c to TPP-IOA or TPP-ISA of 1:20 ( Fig. 5b ). 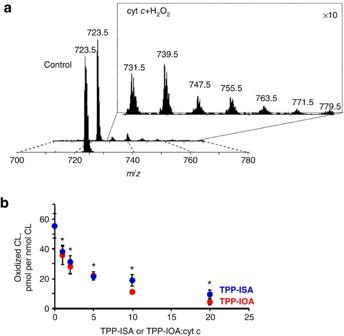Figure 5: Inhibition of H2O2-induced TLCL peroxidation. (a) Typical ESI mass spectra of doubly charged molecular ions of non-oxidized TLCL and TLCL oxidized by CL/cytcand H2O2. Mass-to-charge (m/z; negative MS mode) values of 723.5 and 731.5, 739.5, 747.5, 755.5, 763.5, 771.5 and 779.5 were assigned to molecular clusters of non-oxidized TLCL and TLCL enriched with 1–7 oxygen atoms, respectively. (b) Quantitative assessment of TLCL and its oxidation products by ESI-MS. Data are means±s.d.,n=3, *P<0.05 (ANOVA) versus TLCL/cytc/H2O2. Figure 5: Inhibition of H 2 O 2 -induced TLCL peroxidation. ( a ) Typical ESI mass spectra of doubly charged molecular ions of non-oxidized TLCL and TLCL oxidized by CL/cyt c and H 2 O 2 . Mass-to-charge ( m / z ; negative MS mode) values of 723.5 and 731.5, 739.5, 747.5, 755.5, 763.5, 771.5 and 779.5 were assigned to molecular clusters of non-oxidized TLCL and TLCL enriched with 1–7 oxygen atoms, respectively. ( b ) Quantitative assessment of TLCL and its oxidation products by ESI-MS. Data are means±s.d., n =3, * P <0.05 (ANOVA) versus TLCL/cyt c /H 2 O 2 . Full size image We then employed a model of intrinsic apoptosis induced in mouse embryonic cells by γ-irradiation and assessed several biomarkers of apoptosis. We found that TPP-IOA and TPP-ISA had similar radiation mitigating effects on mouse embryonic cells as evidenced by phosphatidylserine (PS) externalization ( Fig. 6a ), caspase 3/7 activation ( Fig. 6b ) and cyt c release ( Fig. 6c ). In contrast, IEOA or ISA —devoid of a mitochondria-targeting TPP-moiety—exerted no protection against apoptosis in mouse embryonic cells ( Fig. 6d ). To verify that the protective effects were realized during mitochondrial stages of apoptosis, TPP-ISA were added to the in vitro 'caspase activation system' containing S100 fraction from mouse embryonic cells [25] . Caspase activation caused by exogenously added cyt c was completely insensitive to TPP-ISA and TPP-IOA ( Fig. 6e ) thus confirming that anti-apoptotic effects of TPP-IOA and TPP-ISA were realized in mitochondria. Furthermore, the anti-apoptotic activity was neither cell- nor stimulus-specific, as TPP-IOA effectively inhibited apoptosis, induced by a mitochondrial complex I inhibitor, rotenone, in cultured mouse lung endothelial cells ( Fig. 6f ). 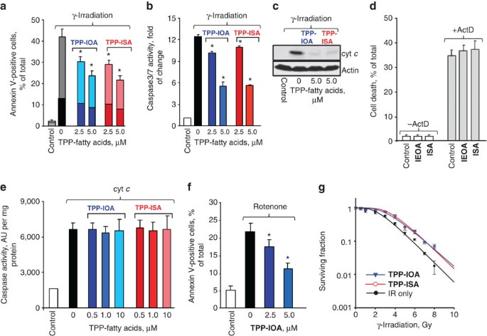Figure 6: Mitigative effects ofTPP-ISAandTPP-IOAagainst apoptosis. Effect ofTPP-ISAandTPP-IOAon γ-irradiation induced PS externalization (dark colour—Annexin V-positive, PI-positive cells; light colour—Annexin V-positive, PI negative cells) (a), caspase 3/7 activation (b), and cytcrelease from mitochondria into the cytosol (anti-cyt c antibody, 0.2 μg ml−1, 1:3,000, Pharmmingen) (c) in mouse embryonic cells. Cells were γ-irradiated to a dose of 10 Gy, and then incubated in the presence of different concentrations ofTPP-ISAorTPP-IOAfor 48 h. Data are means±s.d.,n=3. *P<0.01 (Student'st-test) versus irradiated only cells.TPP-ISAorTPP-IOAwas added to cells 30 min after γ-radiation. (d) Effect ofIEOAandISAon actinomycin D-induced cell death in mouse embryonic cells.IEOAorISAwere incubated in the presence of fatty acid-free bovine serum albumin (BSA) (Sigma) at a molar ratio of 5:1 at 37 °C for 30 min. Mouse embryonic cells were incubated withIEOA/BSA orISA/BSA (100 μM) complexes for 30 min before the addition of 100 ng ml−1actinomycin D (ActD). After 18-h incubation with ActD, cell viability was analysed by flow cytometry using an Annexin V/PI kit. ActD-induced cell death in ~34.2% of cells. Treatment of cells withISAorIEOAin concentrations ranging from 1 to 100 μM exerted no detectable protection against ActD-induced cell death. Representative data with 100 μMIEOA/BSA andISA/BSA complexes are shown. Data are means±s.d.,n=3. (e) Effect ofTPP-ISAandTPP-IOAon caspase-3 activation in S-100 from mouse embryonic cells. Data are means±s.d.,n=3. (f) Effect ofTPP-IOAon mouse lung endothelial cells treated with rotenone (apoptosis was assessed by PS externalization). Data are means±s.d.,n=3. *P<0.05 (Student'st-test) versus rotenone challenged cells. (g) Effect ofTPP-ISAandTPP-IOAon clonogenic survival of mouse embryonic cells after γ-irradiation. The data were fitted to a single-hit multi-target model. Data are means±s.d.,n=3.TPP-IOAorTPP-ISAwas added to cells 30 min after γ-radiation. Figure 6: Mitigative effects of TPP-ISA and TPP-IOA against apoptosis. Effect of TPP-ISA and TPP-IOA on γ-irradiation induced PS externalization (dark colour—Annexin V-positive, PI-positive cells; light colour—Annexin V-positive, PI negative cells) ( a ), caspase 3/7 activation ( b ), and cyt c release from mitochondria into the cytosol (anti-cyt c antibody, 0.2 μg ml −1 , 1:3,000, Pharmmingen) ( c ) in mouse embryonic cells. Cells were γ-irradiated to a dose of 10 Gy, and then incubated in the presence of different concentrations of TPP-ISA or TPP-IOA for 48 h. Data are means±s.d., n =3. * P <0.01 (Student's t -test) versus irradiated only cells. TPP-ISA or TPP-IOA was added to cells 30 min after γ-radiation. ( d ) Effect of IEOA and ISA on actinomycin D-induced cell death in mouse embryonic cells. IEOA or ISA were incubated in the presence of fatty acid-free bovine serum albumin (BSA) (Sigma) at a molar ratio of 5:1 at 37 °C for 30 min. Mouse embryonic cells were incubated with IEOA /BSA or ISA /BSA (100 μM) complexes for 30 min before the addition of 100 ng ml −1 actinomycin D (ActD). After 18-h incubation with ActD, cell viability was analysed by flow cytometry using an Annexin V/PI kit. ActD-induced cell death in ~34.2% of cells. Treatment of cells with ISA or IEOA in concentrations ranging from 1 to 100 μM exerted no detectable protection against ActD-induced cell death. Representative data with 100 μM IEOA /BSA and ISA /BSA complexes are shown. Data are means±s.d., n =3. ( e ) Effect of TPP-ISA and TPP-IOA on caspase-3 activation in S-100 from mouse embryonic cells. Data are means±s.d., n =3. ( f ) Effect of TPP-IOA on mouse lung endothelial cells treated with rotenone (apoptosis was assessed by PS externalization). Data are means±s.d., n =3. * P <0.05 (Student's t -test) versus rotenone challenged cells. ( g ) Effect of TPP-ISA and TPP-IOA on clonogenic survival of mouse embryonic cells after γ-irradiation. The data were fitted to a single-hit multi-target model. Data are means±s.d., n =3. TPP-IOA or TPP-ISA was added to cells 30 min after γ-radiation. Full size image Mitochondria are believed to be involved in orchestration of different cell death pathways [26] , [27] . We found that necrotic cells (propidium iodide (PI)-positive, Annexin V-positive) represented 12.9% while apoptotic cells (PI-negative, Annexin V-positive) were accountable for 28.9% of total PS-positive cells detectable after irradiation. Treatment with TPP-IOA caused a twofold decrease in the number of apoptotic cells (to 14.8%) and 1.6-fold reduction in the number of necrotic cells (to 8.2%). Similarly, TPP-ISA protected via both anti-apoptotic and anti-necrotic mechanisms (to 13.9% of apoptotic and 7.8% necrotic cells, respectively). Overall, these results suggest that PP-IOA and TPP-ISA afforded the radiomitigation in mouse embryonic cells acting through both anti-apoptotic and anti-necrotic pathways. In addition to apoptosis, and necrosis, mitotic cell death can be also triggered in irradiated cells. Using clonogenic assay, that includes the mitotic cell death component, we demonstrated that post-irradiation treatment of mouse embryonic cells with TPP-ISA or TPP-IOA resulted in a significant protection. Using a single-hit multi-target model, we estimated that TPP-ISA or TPP-IOA increased D 0 —the dose needed to reduce cell surviving fraction to 37% (1/ e )—to 1.67±0.06 and 1.71±0.05, respectively, compared with 1.33±0.08 in untreated cells ( Fig. 6g ). Radiomitigative effects of of TPP-IOA and TPP-ISA Given the ability of TPP-IOA and TPP-ISA to act as radiomitigators in vitro , we assessed their potential to act as radioprotectors/radiomitigators in vivo . C57BL/6NTac female mice were exposed to 9.25 Gy total body irradiation at the dose rate of 80 cGy min −1 using the cesium irradiator. Three independent experiments (the total number of mice in each group was 31–35) yielded similar results: irradiation resulted in death of animals within 13–15 days (with survival of only 20% of animals by day 30). TPP-IOA or TPP-ISA (i.p. injection, 5 mg per kg body weight, 10 min after irradiation) showed a strong radiomitigative effect for both compounds ( Fig. 7a ). There was no statistically significant difference in radiomitigative potency of TPP-IOA and TPP-ISA ( P =0.6389, a two-sided log-rank test). We also used a clinical linear accelerator to deliver the radiation dose. The mice (three groups with 22–23 animals in each) were irradiated to 9.25 Gy at the dose rate of 100 cGy min −1 using a Varian TrueBeam linear accelerator (Varian Medical Systems) and injected i.p. with 5 mg per kg body weight of either TPP-ISA or TPP-IOA , 10 min after irradiation. Similarly to the results with cesium irradiator, the survival curves over 52 days were statistically different for TPP-IOA (5 mg per kg body weight) and TPP-ISA (5 mg per kg body weight) versus irradiated controls ( Table 1 ); however, there was no statistically significant difference between TPP-IOA and TPP-ISA ( P =0.4567, a two-sided log-rank test). Thus, after multiple experiments, using two different irradiators, we demonstrated a high potency of both TPP-IOA and TPP-ISA in mitigating radiation damage without significant difference in radiomitigative activity between them. Therefore, all subsequent in vivo experiments were conducted with TPP-IOA and linear accelerator as the radiation source. We chose a dose of 5 mg per kg body weight of TPP-IOA , because a lower dose (2.5 mg per kg body weight) of drug was not effective in mitigating the mice against irradiation. When mice (10 per group) were irradiated and administered 2.5 mg per kg body weight (10 min after irradiation), there was a trend towards a greater survival that, however, did not reach the level of significance ( P =0.0525, a two-sided log-rank test) ( Table 1 ). We further tested whether TPP-IOA was protective if given at later time points (than 10 min) after irradiation (10 mice per group). Administration of TPP-IOA at 5 or 24 h after irradiation resulted in a significant increase in survival ( Fig. 7b , Table 1 ). TPP-IOA was also protective if given 10 min or 1 h before irradiation ( Fig. 7b ; Table 1 ). 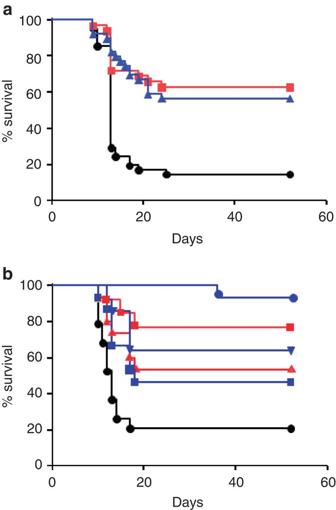Figure 7: Radiation protection and mitigation byTPP-IOAandTPP-ISA. C57BL/6NTac female mice were exposed to total body irradiation to a dose of 9.25 Gy using a cesium source (n=31–35 mice per group) (a) or a linear accelerator (n=10–23 mice per group) (b). (a) The mice were irradiated and injected i.p. withTPP-IOAorTPP-ISA(5 mg per kg body weight in 100 μl of water containing 25% ethanol) 10 min after irradiation. Mice exposed to: total body irradiation at the dose of 9.25 Gy only (black circles); to total body irradiation at the dose of 9.25 Gy and injected withTPP-ISA(5 mg per kg body weight) 10 min (blue triangles) orTPP-IOA(5 mg per kg body weight) 10 min (red squares) thereafter.P<0.0001 (a two-sided log-rank test)—TPP-IOAorTPP-ISAinjected and exposed to total body irradiation mice versus mice exposed to total body irradiation only. (b) The mice were injected i.p. withTPP-IOA(5 mg per kg body weight in 100 μl of water containing 25% ethanol) at 1 h or 10 min before irradiation or 10 min, 5 or 24 h after irradiation. Mice exposed to: total body irradiation at the dose of 9.25 Gy only (black circles); to total body irradiation at the dose of 9.25 Gy and injected withTPP-IOA(5 mg per kg body weight) 10 min (blue circles), 5 h (blue triangles) and 24 h (blue squares) thereafter. Mice injected withTPP-IOA(5 mg per kg body weight) 10 min (red squares) and 1 h (red triangles) before total body irradiation (9.25 Gy). For assessments of significance seeTable 1. Figure 7: Radiation protection and mitigation by TPP-IOA and TPP-ISA . C57BL/6NTac female mice were exposed to total body irradiation to a dose of 9.25 Gy using a cesium source ( n =31–35 mice per group) ( a ) or a linear accelerator ( n =10–23 mice per group) ( b ). ( a ) The mice were irradiated and injected i.p. with TPP-IOA or TPP-ISA (5 mg per kg body weight in 100 μl of water containing 25% ethanol) 10 min after irradiation. Mice exposed to: total body irradiation at the dose of 9.25 Gy only (black circles); to total body irradiation at the dose of 9.25 Gy and injected with TPP-ISA (5 mg per kg body weight) 10 min (blue triangles) or TPP-IOA (5 mg per kg body weight) 10 min (red squares) thereafter. P <0.0001 (a two-sided log-rank test)— TPP-IOA or TPP-ISA injected and exposed to total body irradiation mice versus mice exposed to total body irradiation only. ( b ) The mice were injected i.p. with TPP-IOA (5 mg per kg body weight in 100 μl of water containing 25% ethanol) at 1 h or 10 min before irradiation or 10 min, 5 or 24 h after irradiation. Mice exposed to: total body irradiation at the dose of 9.25 Gy only (black circles); to total body irradiation at the dose of 9.25 Gy and injected with TPP-IOA (5 mg per kg body weight) 10 min (blue circles), 5 h (blue triangles) and 24 h (blue squares) thereafter. Mice injected with TPP-IOA (5 mg per kg body weight) 10 min (red squares) and 1 h (red triangles) before total body irradiation (9.25 Gy). For assessments of significance see Table 1 . Full size image Table 1 TPP-IOA and TPP-ISA increase survival of mice following irradiation. Full size table Given the high radioprotective/radiomitigative activity of TPP-IOA , we determined the extent to which it would be absorbed to reach radiosensitive tissues. This required the development of new LC-MS/MS protocols to quantitate TPP-IOA in tissue samples. These involved the establishment of a selective reaction monitoring protocol for TPP-IOA that provides high selectivity and sensitivity. Our direct assessments clearly demonstrated the presence of TPP-IOA in plasma ( Supplementary Fig. S5 ) as well as in the two most important radiosensitive tissues, bone marrow and small intestine. TPP-IOA levels were highest in plasma (54.0 ng ml −1 of plasma), followed by small intestine (1.5 ng per g of tissue) and bone marrow (0.2 ng per g of tissue), at the 10 min time point after i.p. injection. The levels measured in plasma are consistent with those found for decyl-TPP, a closely related compound, as seen in the study by Porteous et al . [28] We showed that, after intravenous injection, the TPP-compounds are distributed rapidly to various tissues and less than 1% remains in plasma after 15 min. In addition, we assessed the hydrolysis of TPP-IOA in tissues (plasma, bone marrow and small intestine) yielding TPP and non-esterified IOA utilizing two different LC-MS/MS approaches: a selected reaction monitoring method to determine the levels of IOA , a likely hydrolysis product of TPP-IOA , in tissue samples, and multiple reaction monitoring offering extremely high selectivity and sensitivity ( Supplementary Fig. S6 ). Using these approaches, we determined that bone marrow had the least amount of hydrolysis, exhibiting a level of 0.6 ng per g tissue per min of the TPP-propyl hydrolysis product. This was followed by a level of 4.1 ng per g tissue per min and 19.0 ng per g tissue per min of the TPP hydrolysis product in plasma and small intestine, respectively. Simple calculations show that the total amounts of non-hydrolysed TPP-IOA plus hydrolysed ( IOA +TPP) will be significantly (approximately two orders of magnitude) higher than those of the non-hydrolysed compound measured in the small intestine and bone marrow. The importance of this is underscored by our data that both TPP-IOA and IOA are effective inhibitors of peroxidase activity of cyt c /CL complexes ( Fig. 3 ) and CL peroxidation ( Fig. 5 ). In this work, we designed, synthesized and explored a new class of mechanism-based mitochondria-targeted inhibitors that act as strong ligands of iron in complexes of cyt c with CL. The compounds 'lock' the catalytic site of the enzymatic complex, inhibiting its ability to facilitate the development of pro-apoptotic oxidative events, and suppress release of cyt c from mitochondria into the cytosol thus inhibiting apoptotic cell death. We demonstrated that imidazole fatty acids specifically interact with partially unfolded cyt c and not with intact cyt c . Indeed, low-temperature (He) EPR experiments indicate that liganding of haem-iron in cyt c by IOA was dependent on the presence of CL. While it is possible that imidazole fatty acids may interact with other haemoproteins—for example, cytochromes P450 (ref. 16 ) their effects on the oxygenase/peroxidase activity of the haemoproteins might depend on several parameters such as redox potential, haem-coordination state, spin states. Notably, many haemoproteins with peroxidase function—cytochromes P450, myeloperoxidase, cyclooxygenase—do not require anionic (phospho)lipids for their activation. Importantly, TPP-ISA and TPP-IOA exerted strong radoprotective/radiomitigative effects in vivo against lethal doses of irradiation of mice (from 1 h before through 24 h after the irradiation). One can envision two possible applications of our findings in clinical practice. One of them may be associated with the employment of the newly discovered radiomitigators for the treatment of victims of terrorist attacks with nuclear devices as well as individuals inadvertently exposed to irradiation resulting from catastrophic nuclear accidents. Intraperitoneal (i.p.) injections of TPP-IOA and TPP-ISA employed in this study is not the preferred route of drug administration in clinical practice, although it has been used for selected drugs in several disease states [29] , [30] , [31] . It is likely that pharmacologists would have to derive new formulations that could be given orally or as a skin patch. For radiation counterterrorism, a topical or trans-dermal delivery system would be preferred. The second kind of applications may be relevant to organ-specific delivery of TPP-IOA and TPP-ISA to protect normal tissues from ionizing irradiation effects in clinical radiotherapy. Several highly effective chemotherapy drugs are known to interact with ionizing irradiation to promote tumour cell killing, but unfortunately, also exacerbate normal tissue toxicity. Local, tissue-specific delivery of TPP-IOA and TPP-ISA may be also important in amelioration of the toxicity of this combined modality cancer therapy. The design of a pharmacological formulation by which to facilitate delivery of TPP-IOA and TPP-ISA to the oral cavity or oropharynx during radiotherapy of head and neck cancer; to the oesophagus during radiotherapy of non-small cell lung cancer; to the bladder during brachytherapy or fractionated pelvic radiotherapy of endometrial or cervix cancer; and to the rectum, during fractionated radiotherapy of prostate cancer, could provide both normal tissue protection and decreased morbidity for conventional treatment protocols and potentially allow radiation dose-escalation to improve local control. γ-Irradiation is a potent carcinogen by virtue of its ability to cause single- and double-strand DNA breaks [32] —the effect that is also associated with a massive p53-dependent cell death in radiosensitive targets (primary lymphoid organs and intestinal epithelium) leading to acute injury [33] , [34] . Although it is known that p53 acts as a potent and important tumour suppressor [35] , it is believed that this tumour suppressor activity is not directly related to p53's acute pathological response to irradiation-induced systemic genotoxicity [34] . Indeed, there is substantial pharmacological [36] and genetic [34] evidence supporting the notion that temporary and reversible suppression of p53, resulting in massive rescue of cells in radiosensitive tissues, is not associated with an increase in carcinogenicity. Rather, the tumour suppressor activity of p53 is related to activities in cells several days after the irradiation-induced systemic genotoxicity. Thus, p53 inhibitors are expected to represent tissue protective drugs to be used under pathological conditions associated with massive apoptotic cell death [37] . Although p53 inhibitors hold therapeutic promise, their potential applications are limited by the tissue specificity of p53-dependent radiosensitivity. For example, despite the pronounced p53-dependent apoptosis that occurs among epithelial cells of the small intestine after irradiation, clinical gastrointestinal acute radiation syndrome develops independently of p53. Thus, radioprotection of the gastrointestinal tract should be based on p53-independent strategies [38] , possibly other types of apoptosis inhibitors. The current work capitalizes on this principle by utilizing mitochondria-targeted inhibitors of cyt c /CL peroxidase activity— TPP-IOA and TPP-ISA —that demonstrated effectiveness in protecting against radiation-induced apoptosis as well as radioprotective and radiomitigative effects in vivo . The mechanism of radiation mitigation proposed herein will prevent acute radiation sickness while having no impact on p53-mediated tumour suppression. When treatment with the mitochondrial-targeted inhibitors of cyt c is withdrawn, those few cells that have acquired a radiation-induced oncogenic chromosome aberration will be eliminated by p53-mediated apoptosis. This acquired oncogenic stress will be present in these cells for many weeks before tumour onset allowing ample time for p53 to execute its function as a tumour suppressor. This study was aimed at the discovery, rather than the development, of novel mitochondria-targeted radiomitigators and radioprotectors. However, further improvements of structural features and pharmacological characteristics of the proposed inhibitors may lead to an optimized series of radioprotectors and radiomitigators with a broad spectrum of biomedical applications in the biodefense area as well as in radiotherapy of cancer, by achieving increased resistance of normal tissues surrounding the tumour. Animals C57BL/6NTac female mice were anaesthetized with Nembutal (1 mg per 20 gm mouse), irradiated to a total body dose of 9.25 Gy using either a Shepherd Mark 1 Model 68 cesium irradiator at a dose rate of 80 cGy min −1 (31–35 mice per group) or a Varian TrueBeam linear accelerator (Varian Medical Systems) at 100 monitor units or 100 cGy min −1 using 6 MV photons with a 40 cm×40 cm field at 100 SSD (10–23 mice per group). Mice were injected intraperitoneally (i.p.) with 5 mg per kg body weight of TPP-IOA in a 100 μl volume of water containing 25% ethanol at 1 h before irradiation, 10 min before irradiation, 10 min after irradiation, 5 h after irradiation and 24 h after irradiation. Other groups were injected i.p. with 2.5 mg per kg body weight of TPP-IOA or 5 mg per kg body weight of TPP-ISA 10 min after irradiation. The mice were followed for the development of haematopoietic syndrome (at which time they were killed). The health of the non-irradiated mice was unexceptional and no adverse side effects were noticed over the period of study (52 days) after i.p. injection of either TPP-IOA or TPP-ISA (5 mg per kg body weight). The log-rank test was used for three analyses: the comparison of overall survival that is defined as the time from the date of radiation to the date of death for all mice under study; the comparison of short-term survival over the first 20 days, that is, the overall survival count at 20 days; and the comparison of conditional survival in mice surviving 20 or more days, that is, the time from the date of radiation to the date of death for all mice who survived 20 days or longer after radiation. All these comparisons were made between each of the treated groups and the radiation-only control group. All procedures were pre-approved and performed according to the protocols established by the Institutional Animal Care and Use Committee of the University of Pittsburgh. Cells Mouse embryonic cells (courtesy of Dr X. Wang, University of Texas, Dallas) were cultured in DMEM supplemented with 15% FBS, 25 mM Hepes, 50 mg per litre uridine, 110 mg per litre pyruvate, 2 mM glutamine, 1× nonessential amino acids, 50 μM β-mercaptoethanol, 0.5×10 6 U per litre mouse leukaemia inhibitory factor, 100 U per litre penicillin, and 100 mg per litre streptomycin in a humidified atmosphere of 5% CO 2 , 95% air at 37 °C. Mouse lung endothelial cells were obtained as previously described [39] . Briefly, lungs were flushed with HBSS containing 10 U ml −1 heparin, then homogenized and digested in type I collagenase using a gentle MACs dissociator (Miltenyi). Pulmonary endothelial cells were isolated by magnetic beads coated with antibody (rat anti-mouse) to PECAM-1 (BD Pharmingen), and seeded for subculture (passage 1). At approximately passage 2, cells were incubated with fluorescently labelled diacetylated LDL followed by FACS sorting for further purification. The enriched PECAM and diacetylated LDL population was sub-cultured on a collagen/gelatin matrix in 2% O 2 , 5% CO 2 , 93% nitrogen in a Coy Hypoxic Glove Box/Chamber in Opti-MEM (Gibco), 10% FBS, 2 mM glutamine, 0.2% retinal-derived growth factor (Vec Technologies), 10 U ml −1 heparin, 0.1 mM non-essential amino acid supplement (Gibco) and 55 μM β-mercaptoethanol (Counted as passage 3). Cells at passage 4–6 were applied to do the experiments. Phosphatidylserine externalization Phosphatidylserine externalization was determined by Annexin V–FITC apoptosis detection kit (Biovision) according to the manufacturer's instruction. Caspase 3/7 activity Caspase–3/7 activity was measured using a luminescence Caspase–Glo 3/7 assay kit (Promega) according to the manufacturer's instruction. Measurement of cyt c release by western blot analysis Cells were collected after 48 h post-irradiation incubation and resuspended in lysis buffer containing 0.05% digitonin for 4 min on ice. Supernatants were collected after centrifugation for 10 min at 10,000 g . Equal amounts of protein were subject to 15% SDS–PAGE, transferred onto a nitrocellulose membrane, and probed with antibodies against cyt c (clone 7H8.2C12, BD Pharmingen) or actin (Novus) (loading control) followed by horseradish peroxidase-coupled detection. The protein band profile was analysed by densitometry using Labworks image acquisition and analysis software (UVP). Liquid-He EPR measurements of ISA and IEOA liganding Conditions: native cyt c (300 μM), IEOA /cyt c (2:1), TOCL/ IEOA /cyt c (20:2:1), 20 mM HEPES buffer, pH 7.4. Samples (200 μl) were placed in 3 mm o.d. suprasil quartz EPR tubes and frozen in liquid nitrogen for subsequent spectroscopic measurements. X-band (9 GHz) EPR spectra were recorded on a Bruker ESP 300 spectrometer equipped with an Oxford Instruments ESR 910 flow cryostat for ultra-low-temperature measurements. Spectra were recorded at 9.8 G modulation amplitude and 200 μW microwave power. The microwave frequency was calibrated by a frequency counter and the magnetic field was calibrated with a gaussmeter. The temperature was calibrated with carbon–glass resistors (CGR-1-1000) from LakeShore. This instrument and the software (SpinCount) to analyse the EPR spectra were provided by Professor Mike Hendrich, Carnegie Mellon University. Molecular docking The structures of the ligands ISA , IOA , IEOA , IDA , TPP-ISA and TPP-IOA were docked to the partially unfolded structure of horse heart cyt c using the Lamarckian genetic algorithm provided by the Autodock 4.0 software [40] , [41] . The partially unfolded structure of cyt c , where the Met 80 containing loop is displaced was obtained using the molecular dynamics simulation approach as described below. The X-ray crystal structure (Protein Database accession code: 1HRC ) was used as the base structure for performing the MD simulations. The docking procedure used was similar to the studies performed earlier [42] , except for the following changes. A cubic box positioned at x , y , and z 0.032, −0.399, and −0.36, respectively, as the centre was built around the protein with 70×52×54 points and a spacing of 0.375 Å between the grid points was used. A total of 25 genetic algorithm runs were considered in each case with an initial population of 300 and a maximum number of 5,000,000 energy evaluations. The top 25 resulting orientations that have less than or equal to 0.5 Å root mean square deviation were clustered together. The best ligand bound to the partially unfolded cyt c structure in each case was chosen based on lowest energy as well as the conformation where the imidazole group was closest to the haem iron. Molecular dynamics simulation Molecular dynamics simulations were performed using the MD software package NAMD [43] using the VEGA ZZ 2.3.2 (ref. 44 ) package as the user interface. The model structure of horse heart cyt c (PDB ID: 1HRC) was downloaded from the Protein Data Bank, and explicit hydrogens were added using the package VEGA ZZ 2.3.2 (ref. 44 ). A spherical solvent cluster with a radius of 48.5 Å positioned at geometric centre of the protein was built and Cl − ions were added to neutralize the system. This system was energy minimized for 2,000 steps using conjugate gradient method. The energy-minimized structure was slowly heated from 0 to 310 K over a period of 100 ps. Following this, 2 ns molecular dynamics simulation was performed at 310 K to obtain the partially unfolded cyt c structure. Statistics For the in vitro experiments, the results are presented as means±s.d. values from at least three experiments, and statistical analyses were performed by either paired/unpaired Student's t -test or one-way ANOVA. As an exploratory analysis, P -values were not adjusted for multiple comparisons. For the survival data, median survival and its 95% confidence interval were calculated for each group, and the two-sided log-rank test was used to examine the differences between irradiated mice and irradiated mice treated with TPP-ISA or TPP-IOA . In all these tests, a P -value of <0.05 was regarded as significant. How to cite this article: Atkinson, J. et al . A mitochondria-targeted inhibitor of cytochrome c peroxidase mitigates radiation-induced death. Nat. Commun. 2:497 doi: 10.1038/ncomms1499 (2011).